MiR-125a targets effector programs to stabilize Treg-mediated immune homeostasis Although different autoimmune diseases show discrete clinical features, there are common molecular pathways intimately involved. Here we show that miR-125a is downregulated in peripheral CD4 + T cells of human autoimmune diseases including systemic lupus erythematosus and Crohn’s disease, and relevant autoimmune mouse models. miR-125a stabilizes both the commitment and immunoregulatory capacity of Treg cells. In miR-125a-deficient mice, the balance appears to shift from immune suppression to inflammation, and results in more severe pathogenesis of colitis and experimental autoimmune encephalomyelitis (EAE). The genome-wide target analysis reveals that miR-125a suppresses several effector T-cell factors including Stat3, Ifng and Il13. Using a chemically synthesized miR-125a analogue, we show potential to re-programme the immune homeostasis in EAE models. These findings point to miR-125a as a critical factor that controls autoimmune diseases by stabilizing Treg-mediated immune homeostasis. The clinical presentation of any specific autoimmune disease is the culmination of complex interactions between genetics, primary and secondary immune effector mechanisms, and environmental triggers [1] , [2] . Although different autoimmune diseases show discrete clinical features, there are common molecular pathways intimately involved, which ultimately define specific diseases [3] , [4] . Distinct lineages of CD4 + T cells can function to both drive and constrain immune-mediated pathology. While T effector cells are often implicated in multiple autoimmune diseases, Treg cells suppress inflammation and control the development of multiple autoimmune diseases, such as type 1 diabetes, multiple sclerosis and inflammatory bowel disease [5] , [6] , [7] . Foxp3 acts as a lineage specification factor of Treg cells. It binds to multiple genes and plays a dual role as both a transcriptional activator and repressor [8] . Sustained expression of Foxp3 amplifies and stabilizes molecular features of Treg precursor cells. Simultaneously, it represses the molecular features deleterious to Treg cell differentiation or function, thereby preventing deviation of Treg cells into effector T-cell lineages [9] , [10] . The extensive involvement of microRNAs (miRNAs) across human diseases helps to understand the pathogenesis of various ailments and might lead to eventual development of effective therapeutics against these diseases [11] . A subset of miRNAs have shown therapeutic promise and are currently actively pursued either in preclinical or clinical trials [12] , [13] . However, most studies and patents in the miRNA field are related to the treatment of cancer, viral infections, ocular disorders, cardiovascular disorders and neurological disorders. Promising miRNA candidates for therapeutic development in autoimmune diseases are still very limited [12] . In this study, we show that miR-125a is downregulated in peripheral CD4 + T cells of multiple human autoimmune diseases and in relevant mouse models. We further utilize miR-125a-deficient mice and show that miR-125a stabilizes both the commitment and immunosuppressive capacity of Treg cells. Deficiency of miR-125a results in more severe colitis and encephalomyelitis (EAE) pathogenesis. The genome-wide target analysis reveals that miR-125a suppresses several effector T-cell factors such as Stat3, Ifng and Il13. Moreover, a chemically synthesized miR-125a analogue not only contributes to EAE prevention but also alleviates established EAE. Together, our findings demonstrate miR-125a as a critical regulator that stabilizes Treg-mediated immune homeostasis and controls autoimmunity. MiR-125a is downregulated in autoimmune CD4 + T cells CD4 + T-helper cells play a variety of important roles in the development and maintenance of various autoimmune diseases. Our miRNA microarray data showed that miR-125a-5p (named ‘miR-125a’ here) was among top 10 downregulated miRNAs in the splenic CD4 + T cells isolated from MRL/ lpr mouse strain, the most commonly studied mouse model for human lupus at 5 and 16 weeks of age ( Supplementary Fig. 1a,c ), as well as in the splenic CD4 + T cells isolated from different progressive stages of experimental autoimmune EAE, which is a mouse model for human multiple sclerosis ( Supplementary Fig. 1b,d ). MiR-125a was also the most significantly downregulated miRNA among all commonly altered miRNAs in the two sets of microarray data. Moreover, previous studies have shown that downregulation of miR-125a in peripheral T cells is associated with human multiple sclerosis [14] . Therefore, we hypothesized that miR-125a might be a commonly dysregulated miRNA in some human autoimmune diseases. To test the hypothesis, we collected samples from another two different human autoimmune diseases and some mouse models, and confirmed that miR-125a was indeed significantly decreased in disease CD4 + T cells compared with healthy CD4 + T cells. These samples included 22 patients with systemic lupus erythematosus (SLE) versus 20 healthy controls ( Fig. 1a ), 12 patients with Crohn’s disease (CD) versus 14 healthy controls ( Fig. 1b ), myelin olygodendrocyte glycoprotein (MOG)-induced EAE versus controls ( Fig. 1c ) and MRL/ lpr mouse strain versus control mice ( Fig. 1d ). Together, these data suggest that miR-125a may be a commonly downregulated miRNA in multiple human autoimmune diseases and related mouse models. 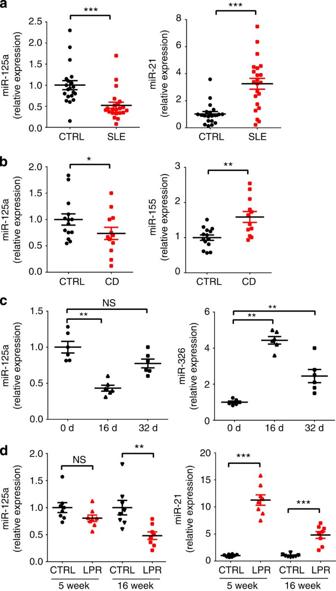Figure 1: MiR-125a is downregulated in autoimmune CD4+T cells. (a) Quantitative realtime (RT)–PCR validation of miR-125a expression, with miR-21 as a positive control, in peripheral CD4+T cells from 22 SLE patients and 20 healthy controls (CTRLs). (b) Quantitative RT–PCR validation of miR-125a expression, with miR-155 as a control, in peripheral CD4+T cells from 12 patients with CD and 14 healthy controls. (c) Quantitative RT–PCR validation of miR-125a expression, with miR-326 as a positive control, in splenic CD4+T cells isolated from six naive control C57BL/6 mice, six EAE mice 16 days after immunization or six EAE mice 32 days after immunization. (d) Quantitative RT–PCR validation of miR-125a expression, with miR-21 as a positive control, in splenic CD4+T cells isolated from MRL/lprmice at 5 or 16 weeks of age and normal controls.n=8 Mice per group. The relative miRNA expression was normalized to the expression of RNU48 (a,b) or snoRNA202 (c,d). All data are mean±s.e.m. *P<0.05, **P<0.01, ***P<0.001 (nonparametric Mann–WhitneyU-test). NS, not significant. Data are representative of two (a,b) or three (c,d) independent experiments. For additional clinical information, refer toSupplementary Tables 1 and 2. Figure 1: MiR-125a is downregulated in autoimmune CD4 + T cells. ( a ) Quantitative realtime (RT)–PCR validation of miR-125a expression, with miR-21 as a positive control, in peripheral CD4 + T cells from 22 SLE patients and 20 healthy controls (CTRLs). ( b ) Quantitative RT–PCR validation of miR-125a expression, with miR-155 as a control, in peripheral CD4 + T cells from 12 patients with CD and 14 healthy controls. ( c ) Quantitative RT–PCR validation of miR-125a expression, with miR-326 as a positive control, in splenic CD4 + T cells isolated from six naive control C57BL/6 mice, six EAE mice 16 days after immunization or six EAE mice 32 days after immunization. ( d ) Quantitative RT–PCR validation of miR-125a expression, with miR-21 as a positive control, in splenic CD4 + T cells isolated from MRL/ lpr mice at 5 or 16 weeks of age and normal controls. n =8 Mice per group. The relative miRNA expression was normalized to the expression of RNU48 ( a , b ) or snoRNA202 ( c , d ). All data are mean±s.e.m. * P <0.05, ** P <0.01, *** P <0.001 (nonparametric Mann–Whitney U -test). NS, not significant. Data are representative of two ( a , b ) or three ( c , d ) independent experiments. For additional clinical information, refer to Supplementary Tables 1 and 2 . Full size image Treg differentiation is defective in miR-125a −/− T cells To further explore the function of miR-125a in autoimmunity, we generated miR-125a transgenic (TG) mice ( Supplementary Fig. 2 ) and knockout (KO) mice ( Supplementary Fig. 3 ). Percentages of T (CD4 + or CD8 + ), B (B220 + ) or myeloid (Mac-1 + ) lineages in peripheral lymph nodes or spleens from 6- to 8-week-old miR-125a KO and control wild-type (WT) mice were initially analysed by flow cytometry. The results showed that there were no statistical differences in these lineages between WT and KO mice ( Supplementary Table. 3 ). We next checked whether miR-125a affected CD4 + T-cell activation or proliferation. Flow cytometric analysis showed that the percentages of different activation markers in CD4 + T ( Supplementary Fig. 4a ) or proliferation of carboxyfluorescein succinimidyl ester (CFSE)-labelled CD4 + T cells ( Supplementary Fig. 4b ) were not significantly altered between KO and WT mice. As a previously reported miRNA profile data have shown that miR-125a was highly expressed in mouse CD4 + CD25 + GITR + Treg cells [15] , we next examined and found that miR-125a was indeed highly expressed in CD4 + CD25 hi population compared with naive T population ( Fig. 2a ) and was also markedly induced in in vitro -derived Treg cell subset ( Fig. 2b ). These data implied that miR-125a might have a function in Treg cells. We further examined the percentages of different T-cell subsets in CD4 + T population from the spleens of KO or WT mice, and found that the proportion and absolute number of Foxp3 + Treg cells showed a significant reduction in miR-125a KO mice compared with that in WT mice ( Fig. 2c–e ), while the other T-cell subsets such as T H 1, T H 2 and T H 17 showed no significant differences ( Supplementary Table. 3 ). To confirm the defective differentiation of Treg in miR-125a-deficient mice, we also sorted naive CD4 + T cells (CD4 + CD25 − CD44 lo CD62L hi ) from 6- to 8-week-old miR-125-deficient mice and their WT littermates, cultured the cells under different T-cell subset-skewing conditions for 4 days and then assessed their differentiation efficiency. Flow cytometric analysis revealed that miR-125a-deficient T cells were indeed impaired in their ability to differentiate into Foxp3 + population compared with WT T cells, even at a high concentration of transforming growth factor (TGF)-β ( Fig. 2f ). Furthermore, the Foxp3 mRNA level was also significantly decreased in miR-125a-deficient Treg cells relative to that in their WT controls ( Fig. 2g ). Consistent with the above in vivo observation, flow cytometric analysis showed miR-125a had no obvious effects on in vitro T H 1, T H 2 and T H 17 differentiation ( Supplementary Fig. 5 ). Together, these results show that miR-125a-deficient T cells may be defective in their ability to differentiate into Treg cells, both in vitro and in vivo . 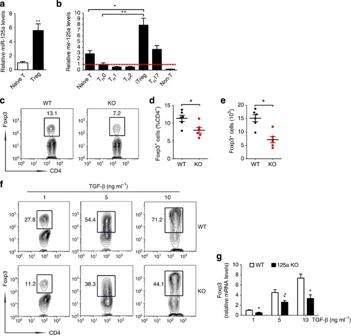Figure 2: Treg differentiation is defective in miR-125a−/−T cells. (a) Naive T cells (CD4+CD25−CD44loCD62hi) and Treg cells (CD4+CD25hi) were isolated from the spleens of C57BL/6 mice. Quantitative RT–PCR analysis of miR-125a expression was performed on these two populations. (b) Quantitative RT–PCR analysis of miR-125a expression in different CD4+T-helper cell subsets differentiatedin vitrofor 4 days under different skewing conditions. (c) Flow cytometric analysis of Foxp3+Treg cells from the spleens of 6- to 8-week-old miR-125a-deficient mice and their WT littermates. (d) Frequency of Foxp3+Treg cells in the CD4+population inc(n=6 per group). (e) Absolute numbers of Foxp3+Treg cells inc(n=6 per group). (f) Flow cytometric analysis of naive CD4+T cells (CD4+CD25−CD44loCD62Lhi) isolated from the spleens of 6- to 8-week-old miR-125a-deficient mice and their WT littermates, cultured for 4 days with IL-2 (5 U ml−1), anti-CD3 antibody (2 μg ml−1) and anti-CD28 antibody (2 μg ml−1), plus various concentrations of TGF-β. (g) Quantitative RT–PCR analysis of Foxp3 expression in Treg cells differentiated as inffrom miR-125a-deficient mice or their WT littermate controls. The relative miR-125a expression was normalized to the expression of snoRNA202 (a,b), while the relative expression levels of Foxp3 were normalized to the expression of mouse Rpl13a. Data are displayed as mean±s.e.m.*P<0.05, **P<0.01 versus control (two-tailed Student’st-test). Data are representative of three (a–f) or four (g) independent experiments. Figure 2: Treg differentiation is defective in miR-125a −/− T cells. ( a ) Naive T cells (CD4 + CD25 − CD44 lo CD62 hi ) and Treg cells (CD4 + CD25 hi ) were isolated from the spleens of C57BL/6 mice. Quantitative RT–PCR analysis of miR-125a expression was performed on these two populations. ( b ) Quantitative RT–PCR analysis of miR-125a expression in different CD4 + T-helper cell subsets differentiated in vitro for 4 days under different skewing conditions. ( c ) Flow cytometric analysis of Foxp3 + Treg cells from the spleens of 6- to 8-week-old miR-125a-deficient mice and their WT littermates. ( d ) Frequency of Foxp3 + Treg cells in the CD4 + population in c ( n =6 per group). ( e ) Absolute numbers of Foxp3 + Treg cells in c ( n =6 per group). ( f ) Flow cytometric analysis of naive CD4 + T cells (CD4 + CD25 − CD44 lo CD62L hi ) isolated from the spleens of 6- to 8-week-old miR-125a-deficient mice and their WT littermates, cultured for 4 days with IL-2 (5 U ml −1 ), anti-CD3 antibody (2 μg ml −1 ) and anti-CD28 antibody (2 μg ml −1 ), plus various concentrations of TGF-β. ( g ) Quantitative RT–PCR analysis of Foxp3 expression in Treg cells differentiated as in f from miR-125a-deficient mice or their WT littermate controls. The relative miR-125a expression was normalized to the expression of snoRNA202 ( a , b ), while the relative expression levels of Foxp3 were normalized to the expression of mouse Rpl13a. Data are displayed as mean±s.e.m. * P <0.05, ** P <0.01 versus control (two-tailed Student’s t -test). Data are representative of three ( a – f ) or four ( g ) independent experiments. Full size image MiR-125a −/− Treg cells fail to prevent colitis effectively We next tried to examine whether there was any defect in the immunoregulatory capacity of Treg cells. To achieve that, we examined Treg cells from miR-125a-deficient and WT mice in overcoming the immune pathogenesis caused by adoptive transfer of naive CD4 + T cells into immunodeficient Rag1 –/– mice. Briefly, naive T cells (CD4 + CD25 − CD44 lo CD62L hi ) were sorted from C57BL/6 WT mice and Treg cells (CD4 + CD25 hi ) were sorted from WT or miR-125a-deficient mice. Then, naive T cells were transferred into Rag1 –/– mice alone or in combination with WT or miR-125a-deficient Treg cells ( Fig. 3a ). Disease progression was assessed by weight loss within 40 days. We observed that Rag1 –/– mice transferred with WT naive T cells alone gradually developed severe body weight loss. Co-transfer of sufficient numbers of WT Treg cells prevented the disease much more effectively than co-transfer of miR-125a-deficient Treg cells, indicating a defect of Treg cell-mediated suppression in miR-125a-deficient mice ( Fig. 3b ). Haematoxylin–eosin staining of the colon sections also showed denser infiltration of leukocytes and more severe epithelial hyperplasia in Rag1 –/– mice co-transferred with miR-125a-deficient Treg cells than those co-transferred with WT Treg cells ( Fig. 3c ). Taken together, these data suggest that miR-125a-deficient Treg cells fail to effectively prevent the immunopathology of T-cell transfer-induced colitis. MiR-125a may contribute to sustain Treg cell-mediated immunosuppressive function. 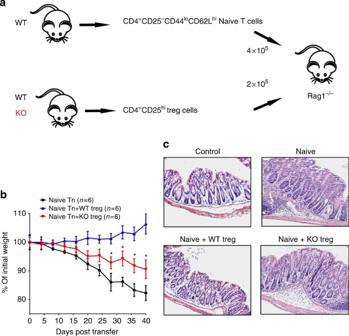Figure 3: MiR-125a−/−Treg cells fail to prevent colitis effectively. (a) Schematic illustration of how T-cell transfer model of colitis was investigated. Each Rag1–/–recipient mouse was transferred with 5 × 105CD4+CD25−CD44loCD62Lhinaive T cells isolated from WT mice, and co-transferred with 2.5 × 105CD4+CD25hiTreg cells isolated from WT or miR-125a-deficient mice. (b) The weight loss of the mice inawas monitored every 4 days for 40 days from the day after injection.n=6 Mice for each group. *P<0.05 (multiple Student’st-test). (c) Representative haematoxylin–eosin staining of colon sections from untreated WT mice (control), Rag1–/–mice transferred with WT naive T cells (naive), Rag1–/–mice co-transferred with WT naive T cells and WT Treg cells (naive+WT Treg), and Rag1–/–mice co-transferred with WT naive T cells and miR-125a-deficient Treg cells (naive+KO Treg; original magnification, × 20). Data are representative of two independent experiments (mean±s.e.m.). Figure 3: MiR-125a −/− Treg cells fail to prevent colitis effectively. ( a ) Schematic illustration of how T-cell transfer model of colitis was investigated. Each Rag1 –/– recipient mouse was transferred with 5 × 10 5 CD4 + CD25 − CD44 lo CD62L hi naive T cells isolated from WT mice, and co-transferred with 2.5 × 10 5 CD4 + CD25 hi Treg cells isolated from WT or miR-125a-deficient mice. ( b ) The weight loss of the mice in a was monitored every 4 days for 40 days from the day after injection. n =6 Mice for each group. * P <0.05 (multiple Student’s t -test). ( c ) Representative haematoxylin–eosin staining of colon sections from untreated WT mice (control), Rag1 –/– mice transferred with WT naive T cells (naive), Rag1 –/– mice co-transferred with WT naive T cells and WT Treg cells (naive+WT Treg), and Rag1 –/– mice co-transferred with WT naive T cells and miR-125a-deficient Treg cells (naive+KO Treg; original magnification, × 20). Data are representative of two independent experiments (mean±s.e.m.). Full size image MiR-125a −/− mice are susceptible to autoimmune EAE To test whether failure to maintain immune homeostasis in the absence of miR-125a was associated with some autoimmune disorders, we induced EAE model in miR-125a-deficient and WT mice. In EAE, Treg cells are required for the suppression of both T H 1- and T H 17-cell subsets [16] . We first evaluated a set of parameters in MOG-induced EAE pathology, and observed that the clinical score and amounts of inflammatory infiltration and demyelination were significantly increased in the miR-125a-deficient mice compared with those in their WT controls ( Fig. 4a,b ). Consistently, the mRNA levels of genes related to T H 1, such as Ifng , and those related to T H 17 lineage, such as Il17a, Il17f, Il21 and Il23r, were significantly upregulated in splenic CD4 + T cell from miR-125a-deficient mice compared with those from WT controls ( Fig. 4c ). The concentration of interferon (IFN)-γ and interleukin-17a (IL-17a) in the supernatants from splenocyte culture challenged with MOG peptide was also increased in miR-125a-deficient mice compared with WT controls ( Fig. 4d ). Furthermore, intracellular cytokine staining showed the percentage of Treg cells in the CD4 + T-cell population isolated from the spleens ( Fig. 4e,f ) and the central nervous system (CNS) infiltrates ( Fig. 4g,h ) were significantly decreased in miR-125a-deficient mice compared with those in the WT controls. In contrast, the percentages of inflammatory IFN-γ- and IL-17a- producing subsets in the CD4 + population were higher in miR-125-deficient mice than that in WT mice in both the spleens ( Fig. 4e,f ) and the CNS infiltrates ( Fig. 4g,h ). Consistently, the clinical score of EAE was lower in the miR-125a TG mice than in WT mice ( Supplementary Fig. 6a ). There were higher levels of in vitro -derived Foxp3 + Treg cells and Foxp3 mRNA in miR-125a TG mice than in WT mice ( Supplementary Fig. 6b,c ). The percentage of IFN-γ + was significantly decreased in the CD4 + T cells isolated from the CNS of TG mice compared with WT mice ( Supplementary Fig. 6d ). Collectively, these experiments show that miR-125a-deficient mice are susceptible to autoimmune EAE, manifesting fewer Treg population and greater production of proinflammatory cytokines in the periphery and CNS. 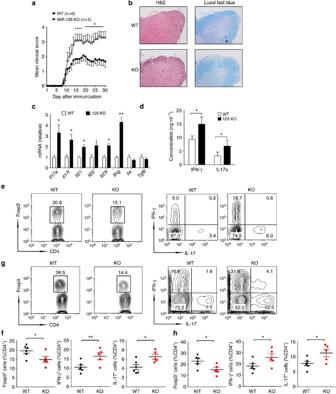Figure 4: MiR-125a−/−mice are susceptible to autoimmune EAE. (a)Mean clinical scores (±s.e.m.) of EAE induced in 6- to 8-week-old WT and miR-125a-deficient mice. (b) Representative haematoxylin–eosin (H&E) staining or Luxol Fast Blue staining of spinal cord sections on day 21 after immunization of the mice ina. (c) Quantitative RT–PCR analysis of gene expression in splenic CD4+T-cell samples on day 21 after immunization of the mice ina. The relative expression levels of different genes were normalized to the expression of mouse Rpl13a. (d) Enzyme-linked immunosorbent assay examination of the concentration of IFN-γ and IL-17a in the supernatants from the splenocyte culture challenged with MOG peptide. (e,g) Representative flow cytometric analysis of the percentage of Treg, TH1 and TH17 cells in the CD4+T cells isolated from the spleens (e) and CNS (g) of the mice (a) on day 21 after immunization. (f,h) The percentages of Foxp3+Treg cells, IFN-γ+T cells and IL-17+T cells in the CD4+populations from the spleens (e) and CNS (g), respectively. *P<0.05, **P<0.01 versus control (two-tailed Student’st-test). Data are representative of three (a,b,e–h) or four (c,d) independent experiments (mean±s.e.m.). Figure 4: MiR-125a −/− mice are susceptible to autoimmune EAE. ( a )Mean clinical scores (±s.e.m.) of EAE induced in 6- to 8-week-old WT and miR-125a-deficient mice. ( b ) Representative haematoxylin–eosin (H&E) staining or Luxol Fast Blue staining of spinal cord sections on day 21 after immunization of the mice in a . ( c ) Quantitative RT–PCR analysis of gene expression in splenic CD4 + T-cell samples on day 21 after immunization of the mice in a . The relative expression levels of different genes were normalized to the expression of mouse Rpl13a. ( d ) Enzyme-linked immunosorbent assay examination of the concentration of IFN-γ and IL-17a in the supernatants from the splenocyte culture challenged with MOG peptide. ( e , g ) Representative flow cytometric analysis of the percentage of Treg, T H 1 and T H 17 cells in the CD4 + T cells isolated from the spleens ( e ) and CNS ( g ) of the mice ( a ) on day 21 after immunization. ( f , h ) The percentages of Foxp3 + Treg cells, IFN-γ + T cells and IL-17 + T cells in the CD4 + populations from the spleens ( e ) and CNS ( g ), respectively. * P <0.05, ** P <0.01 versus control (two-tailed Student’s t -test). Data are representative of three ( a , b , e–h ) or four ( c , d ) independent experiments (mean±s.e.m.). Full size image MiR-125a −/− Treg cells display increased effector T genes To gain insights into the general functional features of miR-125a-deficient Treg cells, we sorted CD4 + CD25 hi Treg population from the spleens of 6- to 8-week-old miR-125a-deficient and their littermate WT mice, and then performed a genome-wide gene-array analysis. We then predicted the biological functions and mapped the biomolecular networks of the differentially expressed gene transcripts using Ingenuity Pathway Analysis tool. The most significant enrichment of the differentially expressed genes was related to T-helper cell pathways. A salient characteristic of Treg cells is their inability to produce proinflammatory cytokines. However, in the absence of miR-125a, Treg cells showed increased expression of genes related to T H 1-, T H 2- and T H 17 subsets, including some lineage-specific transcriptional factors, cytokines and cytokine receptors. Consistently, Treg lineage-specific transcription factor Foxp3 was decreased, together with some cytokine genes such as Tgfb1 ( Fig. 5a ). We further examined the expression of most of the genes cited above with real-time PCR. The results confirmed the array data ( Fig. 5b ), showing that in the absence of miR-125a, Treg cells showed increased expression of effector lineage genes and reduced expression of Treg lineage genes such as Foxp3. These data also implied that sustained expression of miR-125a in Treg cells may restrain the differentiation programs of effector lineages to stabilize Treg lineage commitment. Although deficiency of miR-125a in Treg cells upregulated T H 1-, T H 2- and T H 17-related genes, miR-125a had no obvious effects on in vitro T H 1, T H 2 and T H 17 differentiation, as well as in vivo proportions of these T effector subsets. Therefore, we postulated that the exaggerated proinflammatory cytokine production in miR-125a-deficient mice at pathogenesis conditions such as EAE might be mainly attributable to the break of immune tolerance caused by reduced differentiation or suppressor function of Treg cells, but might not be a cell-intrinsic property of miR-125a-deficient effector T cells. 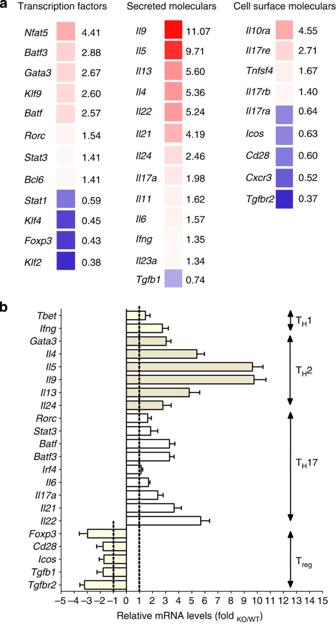Figure 5: MiR-125a−/−Treg cells display increased effector T genes. (a) Genome microarray analysis of CD4+CD25hiTreg cells from miR-125a-deficient and WT mice. Splenic CD4+T cells from miR-125a-deficient and WT mice were enriched by Miltenyi Biotec beads. Then, Treg cells (CD4+CD25hi) were sorted by flow cytometry and harvested in Trizol. Samples from three independent experiments were pooled for the microarray analysis. Ingenuity Pathway Analysis analysis was used to investigate which molecular pathways were affected by miR-125a deficiency. Genes that are associated with the T-helper cell pathways show the most significant enrichment, among which gene transcripts up- or downregulated by >30% are listed ina. Left, gene symbols. Right, fold change of gene expression in miR-125a-deficient Treg compared with WT Treg. (b) Quantitative RT–PCR analysis of the expression levels of genes associated with T-helper cell differentiation pathway ina. Different T-helper cell subsets are marked in different colours. Data are representative of three (b) independent experiments (mean±s.e.m.). Array data are available in GEO under accession codeGSE66608. Figure 5: MiR-125a −/− Treg cells display increased effector T genes. ( a ) Genome microarray analysis of CD4 + CD25 hi Treg cells from miR-125a-deficient and WT mice. Splenic CD4 + T cells from miR-125a-deficient and WT mice were enriched by Miltenyi Biotec beads. Then, Treg cells (CD4 + CD25 hi ) were sorted by flow cytometry and harvested in Trizol. Samples from three independent experiments were pooled for the microarray analysis. Ingenuity Pathway Analysis analysis was used to investigate which molecular pathways were affected by miR-125a deficiency. Genes that are associated with the T-helper cell pathways show the most significant enrichment, among which gene transcripts up- or downregulated by >30% are listed in a . Left, gene symbols. Right, fold change of gene expression in miR-125a-deficient Treg compared with WT Treg. ( b ) Quantitative RT–PCR analysis of the expression levels of genes associated with T-helper cell differentiation pathway in a . Different T-helper cell subsets are marked in different colours. Data are representative of three ( b ) independent experiments (mean±s.e.m.). Array data are available in GEO under accession code GSE66608 . Full size image Mir-125a inhibits several effector T lineage factors The above results raised several questions such as how exactly miR-125a restrained effector lineage programs in Treg cells, and whether the elevated genes in miR-125-deficient Treg cells were the direct targets of miR-125a or the consequence of a secondary effect caused by the reduced expression of Foxp3. To answer these questions, we screened the direct targets of miR-125a by combining target prediction by TargetScan with microarray gene expression data to identify the overlapping and upregulated gene transcripts. Using a combination of these two approaches, we identified 74 genes. Among them, only five predicted genes ( Stat3, Tnfsf4, Tnfaip3, Mapkapk2 and Ppp5c ) have been reported to have the potential functions in immune responses or pathways ( Supplementary Table 4 ). We confirmed the inhibitory effect using a luciferase reporter assay and found that miR-125a significantly suppressed the luciferase activity of the 3′ untranslated region (UTR) of Stat3 and Tnfsf4 ( Supplementary Fig. 7 ). To avoid potentially significant miR-125a targets from being excluded, we next examined the genes that belonged to T-helper cell pathway and whose expression were inversely correlated to the expression of miR-125a in the array data, including those encoding major transcription factors, cytokines, cytokine receptors and signalling molecules, and focused on 21 potential genes ( Supplementary Table 5 ). We next cloned the 3′UTRs of all these genes into luciferase reporter constructs, and found that miR-125a markedly repressed the reporter activities of several genes, including Stat3 , Il13 and Ifng , whereas the activity of others was either slightly affected or unaffected by miR-125a ( Fig. 6a ). We further identified the potential binding sites of miR-125a in the 3′UTRs of Stat3, Il13 and Ifng by TargetScan ( Fig. 6b ). Mutation of these binding sites confirmed the suppressive roles of miR-125a on these genes ( Fig. 6c ). To further demonstrate that Stat3, Il13 and Ifng were the direct targets of miR-125a, we next detected the relative mRNA and protein levels of the targets after overexpression of miR-125a. Since Stat3 is constitutively expressed in some human and mouse cell lines, and the target sites are highly conserved between different species, we first transfected HEK293T cells with two different doses of miR-125a agomirs that are chemically synthesized double-stranded RNA (dsRNA) oligonucleotides used to mimic miRNA. We also infected mouse CD4 + T cells with retrovirus-mediated overexpression of miR-125a. The results that showed miR-125a suppressed the protein levels of endogenous Stat3 expression in a dose-dependent manner ( Fig. 6d ). Considering Il13 and Ifng are secreted cytokines, we next generated retrovirus-based constructs to overexpress miR-125a, and infected CD4 + T cells under Th1- or Th2-skewing conditions for 4 days, respectively. The infection efficiency, calculated as the percentage of GFP + cells, was ∼ 40% when the cells were infected once, and >85% when they were infected repeatedly ( Supplementary Fig. 8 ). The amounts of IFN-γ and IL-13 in the supernatants of the cells infected with miR-125a were significantly reduced compared with that in cells infected with the empty vector ( Fig. 6e ). The mRNA levels of Stat3, Ifng and Il13 were also significantly reduced after overexpression of miR-125a ( Fig. 6f ). Considering the fact that Stat3 is a critical transcriptional factor required for T H 17 differentiation, which inhibits Smad3 binding to enhancer I to limit Treg differentiation [17] , [18] , Ifng and Il13 are T H 1/T H 2 polarizers that can also potently inhibit Foxp3 expressing Treg cells differentiation from naive CD4 + precursors [19] , [20] , these data therefore show that miR-125a directly represses several targets of effector T lineages that are detrimental to Treg differentiation, which may help to stabilize Treg lineage commitment and function. 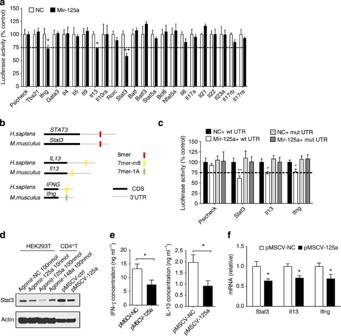Figure 6: Mir-125a inhibits several effector T lineage factors. (a) MiR-125a targets Stat3, Il13 and Ifng. Dual luciferase assay of HEK293T cells co-transfected with reporter vectors containing the 3′UTRs of different genes and miR-125a agomir or control agomir. The renilla luciferase activity was normalized to the Firefly luciferase activity. Data are shown as relative luciferase activities of cells transfected with miR-125a related to those of the control cells. (b) Comparison of miR-125a-responsive elements in human and mice transcripts encoding Stat3 (STAT3 and Stat3, respectively), Il13 (IL13 and Il13, respectively) and Ifng (IFNGandIfng, respectively) by TargetScan. Colours in the key indicate branch lengths (and match to miR-125a). CDS, coding sequence. (c) Dual luciferase assay of HEK293T cells co-transfected the indicated WT or point-mutated 3′UTR-driven reporter constructs (wt UTR or mut UTR, respectively) with miR-125a or control agomirs. (d) Western blotting of endogenous STAT3 protein levels after transfection of HEK293T cells or infection of CD4+T cells with different doses of miR-125a agomirs or miR-125a retrovirus for 2 days. MiR-148a was used as a control. (e) Enzyme-linked immunosorbent assay examination of IFN-γ and IL-13 in the supernatants of CD4+T cells transfected with retrovirus-based miR-125a or empty vector, and differentiated under TH1- or TH2-skewing conditions for 4 days. (f) Quantitative RT–PCR analysis of the mRNA levels of Stat3, Il13 and Ifng after the retrovirus-based overexpression of miR-125a in CD4+T cells for 4 days. The relative expression levels were normalized to the expression of mouseRpl13a.Data are representative of four (a) or three (c–f) independent experiments (mean±s.e.m.). *P<0.05, **P<0.01 versus control (two-tailed Student’st-test;a,e,f) or (one-way analysis of variance and least significant differencet-test;c). Figure 6: Mir-125a inhibits several effector T lineage factors. ( a ) MiR-125a targets Stat3, Il13 and Ifng. Dual luciferase assay of HEK293T cells co-transfected with reporter vectors containing the 3′UTRs of different genes and miR-125a agomir or control agomir. The renilla luciferase activity was normalized to the Firefly luciferase activity. Data are shown as relative luciferase activities of cells transfected with miR-125a related to those of the control cells. ( b ) Comparison of miR-125a-responsive elements in human and mice transcripts encoding Stat3 ( STAT3 and Stat3 , respectively), Il13 ( IL13 and Il13 , respectively) and Ifng ( IFNG and Ifng , respectively) by TargetScan. Colours in the key indicate branch lengths (and match to miR-125a). CDS, coding sequence. ( c ) Dual luciferase assay of HEK293T cells co-transfected the indicated WT or point-mutated 3′UTR-driven reporter constructs (wt UTR or mut UTR, respectively) with miR-125a or control agomirs. ( d ) Western blotting of endogenous STAT3 protein levels after transfection of HEK293T cells or infection of CD4 + T cells with different doses of miR-125a agomirs or miR-125a retrovirus for 2 days. MiR-148a was used as a control. ( e ) Enzyme-linked immunosorbent assay examination of IFN-γ and IL-13 in the supernatants of CD4 + T cells transfected with retrovirus-based miR-125a or empty vector, and differentiated under T H 1- or T H 2-skewing conditions for 4 days. ( f ) Quantitative RT–PCR analysis of the mRNA levels of Stat3, Il13 and Ifng after the retrovirus-based overexpression of miR-125a in CD4 + T cells for 4 days. The relative expression levels were normalized to the expression of mouse Rpl13a. Data are representative of four ( a ) or three ( c–f ) independent experiments (mean±s.e.m.). * P <0.05, ** P <0.01 versus control (two-tailed Student’s t -test; a , e , f ) or (one-way analysis of variance and least significant difference t -test; c ). Full size image MiR-125a agomir treatment ameliorates EAE pathogenesis A series of studies have supported the systemic administration of miRNA as a therapeutic strategy [21] , [22] . Our current studies showed the suppressive roles of miR-125a on the pathogenesis of autoimmune animal models. Therefore, we sought to evaluate the efficacy and potential application of a miR-125a-based therapy for autoimmune pathogenesis, such as EAE. Agomirs or antagomirs are synthetic RNA molecules with improved stability and delivery, and have been shown to achieve therapeutic overexpression or silencing of an endogenous miRNA gene in vivo [23] , [24] . To confirm the efficacy of a systemic administration of miR-125a agomir or antagomir in vivo , we first injected mice intravenously with miR-125a agomir, antagomir or their corresponding controls. Different tissues were collected 24 h after the injection, and miR-125a expression was determined by quantitative PCR. The results showed that miR-125a can be efficiently overexpressed or silenced in most tissues, including the liver, kidney and spleen, but not in the brain, suggesting that agomirs and antagomirs minimally cross the blood–brain barrier ( Supplementary Fig. 9 ). We also used florescence-labelled miR-125a agomirs to show the systemic transfection efficiency of miRNA into CD4 + T cells. Cy5-labelled miR-125a agomirs was first transfected into CD4 + T cells in vitro , and confocal microscopy image showed that the Cy5 fluorescence label was successful ( Supplementary Fig. 10a ). Cy5-labelled agomirs were further intravenously injected into WT mice for continuous 3 days, and the lymphocytes were harvested 1 day later to test the transfection efficiency. Flow data showed that the transfection efficiency of Cy5-labelled agomir into CD4 + T cells in vivo was ∼ 58% in lymph nodes and 53% in spleen after three injections ( Supplementary Fig. 10b ). Since miR-125a sustains Treg cell differentiation and suppressive function during the pathogenesis of EAE, we postulated that treatment with miR-125a agomir could ameliorate the pathogenesis of EAE. As expected, after intravenously injecting a high dose of miR-125a agomir three times at the onset of EAE (within 1 day of initial symptoms), the disease severity was markedly reduced, accompanied by decreased CNS inflammation and demyelination ( Fig. 7a,b ). Consistently, the percentage of Treg cells was significantly increased (11.6±1.08% versus 18.7±1.59%; P <0.01; Fig. 7c ), whereas the percentage of IFN-γ + (28.8±2.82% versus 20.7±2.07%, respectively; P <0.05) and IL-17 + proinflammatory subsets (12.8±1.06% versus 8.9±1.05%, respectively; P <0.05) were significantly decreased in the CD4 + T cells isolated from the CNS after treatment with miR-125a agomirs ( Fig. 7d–f ). In contrast, the disease severity of EAE increased significantly with the antagomir-mediated silencing of miR-125a at the onset of EAE ( Supplementary Fig. 11 ), which is consistent with the results of miR-125a-deficient mice. Moreover, to test the role of miR-125 in a therapeutic approach in EAE [25] , [26] , we also administered miR-125a agomir for continuous 3 days after acute EAE was established, at a clinical score 1–2. The results showed that miR-125a agomir treatment also significantly ameliorated established EAE symptoms ( Fig. 7g and Supplementary Fig. 12 ). Taken together, these data suggest that manipulation of miR-125a expression in vivo not only contributed to EAE prevention but also alleviated established EAE. 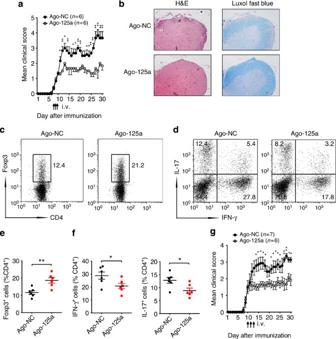Figure 7: MiR-125a agomir treatment ameliorates EAE pathogenesis. (a) Mean clinical scores (±s.e.m.) for EAE induced in 6- to 8-week-old WT mice after three intravenous (i.v.) injections of miR-125a agomir or control agomir (5 μ mol kg−1per day per mouse) at the onset of EAE. (b) Representative haematoxylin–eosin (H&E) staining or Luxol Fast Blue staining of spinal cord sections on day 21 after immunization of the mice ina. (c) Flow cytometric analysis of the percentage of Treg cells in the CD4+T cells isolated from the CNS of the mice inaon day 21 after immunization. (d) Flow cytometric analysis of the percentages of TH1 and TH17 in the CD4+T cells isolated from the CNS of the mice (a) on day 21 after immunization. (e) Mean percentages (±s.e.m.) of Foxp3+Treg cells in the CD4+population ofc(n=6 per group). (f) Mean percentages (±s.e.m.) of IL-17+or IFN-γ+T cells in the CD4+population ofd(n=6 per group). (g) Mean clinical scores (±s.e.m) for EAE induced in 6- to 8-week-old WT mice with three injections of miR-125a agomir (5 μ mol kg−1per day per mouse) after acute EAE was established, at a clinical score 1–2.n=7 or 6 per group. The EAE symptoms were evaluated every day. Data are representative of three (a) or two (c–g) independent experiments (mean±s.e.m.). *P<0.05, **P<0.01 (two-tailed Student’st-test). Figure 7: MiR-125a agomir treatment ameliorates EAE pathogenesis. ( a ) Mean clinical scores (±s.e.m.) for EAE induced in 6- to 8-week-old WT mice after three intravenous (i.v.) injections of miR-125a agomir or control agomir (5 μ mol kg −1 per day per mouse) at the onset of EAE. ( b ) Representative haematoxylin–eosin (H&E) staining or Luxol Fast Blue staining of spinal cord sections on day 21 after immunization of the mice in a . ( c ) Flow cytometric analysis of the percentage of Treg cells in the CD4 + T cells isolated from the CNS of the mice in a on day 21 after immunization. ( d ) Flow cytometric analysis of the percentages of T H 1 and T H 17 in the CD4 + T cells isolated from the CNS of the mice ( a ) on day 21 after immunization. ( e ) Mean percentages (±s.e.m.) of Foxp3 + Treg cells in the CD4 + population of c ( n =6 per group). ( f ) Mean percentages (±s.e.m.) of IL-17 + or IFN-γ + T cells in the CD4 + population of d ( n =6 per group). ( g ) Mean clinical scores (±s.e.m) for EAE induced in 6- to 8-week-old WT mice with three injections of miR-125a agomir (5 μ mol kg −1 per day per mouse) after acute EAE was established, at a clinical score 1–2. n =7 or 6 per group. The EAE symptoms were evaluated every day. Data are representative of three ( a ) or two ( c–g ) independent experiments (mean±s.e.m.). * P <0.05, ** P <0.01 (two-tailed Student’s t -test). Full size image The extensive involvement of miRNAs across human diseases helps to understand the pathogenesis of various ailments and lead to therapeutics. However, the promising miRNA candidates for controlling autoimmune pathogenesis are still limited. Our previous work has that shown miR-125a is downregulated in the peripheral CD3 + T cells of SLE patients [27] . Interestingly, miR-125a was also downregulated in oral lichen planus, which is a T-cell-mediated autoimmune disease of oral mucosa [28] . In this study, we further identified miR-125a as a commonly downregulated miRNA in peripheral CD4 + T cells of multiple human autoimmune diseases such as SLE and CDs, as well as their related animal disease models. These findings thus provided a very valuable candidate with potential as a biomarker of some autoimmune diseases. Furthermore, we identified miR-125a as a regulator that stabilizes the commitment and immunoregulatory capacity of Treg cells by restraining the differentiation programs of other effector lineages, consequently for the suppression of inflammation. This finding identified miR-125a as a key regulator of CD4 + T-cell differentiation that prevents autoimmune pathogenesis by controlling the balance between tolerance and autoimmunity. During the early stage of T-cell differentiation, the cells potentially integrate different environment clues and ultimately allow cells to move towards committing to a particular T-cell lineage [29] , [30] . The fate decision involves the competition of various transcription factors that dictate different T-cell differentiation programs [31] , [32] , [33] . Recent studies regarding Treg cells development suggests that the decision of antigen-stimulated cells to differentiate into different T cells subtypes may depend on balancing polarizing cytokines regulated by T cells subtype-specific transcription factors [32] , [34] . It has been shown that Foxp3 and Gata3, a specific T H 2 transcription factor, are able to physically associate with each other to determine T-cell differentiation to either Treg or T H 2 (ref. 35 ). Similarly, interaction between Foxp3 and Rorc appears to reciprocally regulate the induction of Treg and T H 17 cells [36] , [37] , [38] . Foxp3 is able to stabilize the molecular features of the Treg lineage and inhibit effector T-cell developmental factors [10] , [39] , [40] . In this study, in the absence of miR-125a, Treg cells showed increased expression of T H 1-, T H 2- and T H 17-related effector lineage genes, as well as reduced expression of Treg lineage genes such as Foxp3 . As such, miR-125a appears to operate as a crucial regulator in modulating the fate decision of Treg lineage and in the maintenance of immune homeostasis. Further target screen demonstrated that miR-125a directly suppressed several targets, including Stat3, Il13 and Ifng, which are critical factors of effector lineages and also detrimental to Treg differentiation. Thus, miR-125a exerts its roles in a manner partially similar to Foxp3. This finding not only explains how sustained expression of miR-125a in Treg cells is required for restraining effector lineage programs to stabilize Treg lineage commitment and function at a molecular level but also provides insights into the mechanism of miR-125a in controlling immune homeostasis in the context of autoimmunity. However, although deficiency of miR-125a upregulates some lineage-specific transcriptional factors, cytokines and cytokine receptors in Treg cells, we did not observe obvious effects of miR-125a on T H 1, T H 2 and T H 17 differentiation. The potential mechanism may be attributable to the following factors: (1) miR-125a is induced and highly expressed in Treg cells but not in effector T cells, so it is probably that only loss function of miR-125a in Treg cells has obvious effects; (2) miR-125a may inhibit other potential targets that have not been identified yet. miR-125a might have a combinational effect on effector T-cell differentiation, and probably happen to target some negative regulators of T H 1 and T H 17 differentiation, in addition to targeting the positive regulators such as Stat3 and IFN-γ. Nevertheless, although the absence of miR-125a expression was not associated with a modulation of T H 2 differentiation in vitro and in vivo on normal conditions, it might be also interesting to test the influence of miR-125a in Th2-prone models such as asthma, in addition to EAE model. Moreover, as we only observed the upregulation of the transcripts of some lineage-specific transcriptional factors, cytokines and cytokine receptors in Treg cells, it also raised a question to measure protein expression of these genes. As Treg cells usually express very low levels of inflammatory cytokines at basal level, a better way is to cross miR-125a KO mice with reporter mice such as Foxp3-Red fluorescent protein (RFP), IL-17-green fluorescent protein (GFP) or IFN-γ-yellow fluorescent protein (YFP) reporter mice. In that case, the relative expression levels of Foxp3 and effector cytokines such as IL-17 and IFN-γ can be easily monitored by the fluorescence intensity of RFP, GFP or YFP under different conditions, such as inflammatory environments. Although previous studies have shown that several miRNAs, such as miR-146a (ref. 41 ), miR-155 (ref. 42 ) and miR-10a (ref. 43 ), regulate Treg cells development, suppressor function or homeostasis, the expression patterns of these miRNAs in different autoimmune diseases are still unclear. Our study demonstrated that miR-125a is a commonly dysregulated miRNA in peripheral CD4 + T cells of multiple human autoimmune diseases and animal models. Although the exact mechanisms for the dysregulation of miR-125a in autoimmune pathogenesis are still unknown, we postulate that there might be a potential possibility involved. Previous works have shown that a single-nucleotide polymorphism is located within the precursor (+8) of the mature miR-125a, which significantly blocks the processing of pri-miRNA to pre-miRNA [44] . Whether the genetic polymorphisms within this single locus are associated with numerous autoimmune diseases might be worth further exploring. Despite the recent discovery of miRNAs, several candidates have already progressed into clinical/preclinical development. The most clinically advanced miRNA-based therapy at the present time is a miR-122 antagonist, SPC3649, that targets an infectious disease—hepatitis C virus—and is currently being evaluated in phase 2 clinical trials [45] , [46] , [47] . Other miRNAs currently in development are in the area of cardiovascular disease and include miR-208 (ref. 48 ), miR-195 and so on. Our work showed that miR-125a agomir not only contributes to EAE prevention but also alleviates established EAE, thus providing very valuable promise for pharmacological intervention of miR-125a in autoimmune diseases. Although the systemic injection of miR-125a agomir for consecutive three times obtained transfection efficiency ∼ 58% in lymph nodes and 53% in spleen, the therapeutic effect of mir-125a agomir on EAE model was quite efficient. One possible reason is that once miR-125a agomir is overexpressed in T cells, it promotes the differentiation of Treg cells and stabilizes Treg commitment and function, therefore altering the ratio of Treg to T effector cells in vivo . Treg cells further produce large amount of cytokines such as TGF-β, which subsequently upregulates miR-125a expression in more CD4 + T cells ( Supplementary Fig. 13 ). Under this condition, mir-125a functions as an initiator and promotes the balance to shift from inflammation to immune suppression through a positive feedback loop. In summary, our study demonstrates miR-125a as a critical factor that controls autoimmune diseases through stabilizing Treg-mediated immune homeostasis by targeting effector programs. And this finding also provides insights into developing potential miRNA-based therapies in autoimmunity. Mice MiR-125a KO mice were generated by replacing a 630-bp-long genome DNA fragment that only encodes mmu-miR-125a with a neomycin selection cassette. The mice were created on the C57BL/6 background by Shanghai Biomodel Organism Science and Technology Development Co., Ltd. The primer sequences used for genotyping were as follows: sense primer 5′-CTGAGGTCTGGATCTCTGGC-3′ and antisense primer 5′-GCTCAGAAACCCAGTGTCACA-3′ for WT mice; sense primer 5′-CTGAGGTCTGGATCTCTGGC-3′ and antisense primer 5′-GCTCAGAAACCCAGTGTCACA-3′ for KO mice. The mice were crossed with Flp mice to get rid of neomycin gene. Six- to 12-week-old miR-125a KO mice and their littermate controls were used for experiments. To generate miR-125a TG (miR-125 TG) mice, a 352-bp-long genome DNA fragment encoding mmu-miR-125a was cloned into the plasmid pSuper, using the forward primer: 5′-TCCCTCTTATTCTGGCTTTCTA-3′ and reverse primer: 5′-GAGGTCAGGTTTCAGTTGGTG-3′. The mice were created on the C57BL/6 background by Shanghai Biomodel Organism Science and Technology Development Co., Ltd. The primer sequences used for genotyping were as follows: sense primer 5′-GTAAAACGACGGCCAGT-3′ and antisense primer 5′-AACAGCTATGACCATG-3′ on the mouse miR-125a-coding sequence. Six- to 12-week-old miR-125a KO or TG mice and their littermate controls were used for experiments. C57BL/6 WT mice were purchased from Shanghai Laboratory Animal Center, Chinese Academy of Sciences. Rag1 −/− mice were purchased from Model Animal Research Center of Nanjing University. All mice were maintained in specific pathogen-free conditions. All animal experiments were performed in compliance with the guide for the care and use of laboratory animals, and were approved by the institutional biomedical research ethics committee of the Shanghai Institutes for Biological Sciences (Chinese Academy of Sciences). Subjects A total of 34 patients (22 SLE patients and 12 CD patients) were included in the study. Thirty-four normal subjects were matched with the patients for age, sex and race. All participants are from Chinese Han population. The participants with concurrent infections were excluded from the study. For additional clinical information, refer to Supplementary Tables 1 and 2 . The study was approved by the Research Ethics Board of Renji Hospital. Peripheral blood samples were collected from each subject in tubes containing acid citrate dextrose formula A. miRNA and DNA microarray Total RNA was isolated using TRIzol reagent (Invitrogen). RNA quality was assessed with an Agilent 2100 Bioanalyzer (Agilent), and only samples with an RNA integrity number >8 were used. For the miRNA expression analysis, a TaqMan Low Density Array v3.0 (Applied Biosystems) was used to detect and quantified up to 754 human miRNAs or 641 mouse miRNAs using an Applied Biosystems real-time instrument, according to the manufacturer’s protocol. Global mRNA expression in iTreg samples from miR-125a-deficient and WT mice were assayed with the Affymetrix GeneChip Mouse Genome 430 2.0 Array. Data were further analysed with Agilent GeneSpring GX 10 Microarray Data Analysis Software. Array data are available in GEO under accession code GSE66608 . Reagents The following antibodies were purchased from BD Pharmingen: anti-mouse CD4–FITC (GK1.5; used at 1:100 dilution), anti-mouse CD25–APC (PC61; used at 1:200 dilution), anti-mouse CD62L–PE (MEL-14; used at 1:200 dilution), anti-mouse CD44–PE/Cy5 (IM7; used at 1:200 dilution), anti-mouse IFN-γ–APC (XMG1.2; used at 1:100 dilution) and anti-mouse IL-17–PE (TC11-18H10; used at 1:100 dilution). The following antibodies were purchased from eBioscience: anti-mouse CD3e Functional Grade Purified (145-2C; final concentration used at 2 μg ml −1 ), anti-mouse CD28 Functional Grade Purified (37.51; final concentration used at 2 μg ml −1 ), anti-mouse/rat Foxp3–PE (FJK-16S; used at 1:100 dilution) and antibody against Stat3 (sc-482; Santa Cruz; used at 1:1,000 dilution). T-cell purification and activation Naive CD4 + CD25 − CD44 lo CD62L hi T cells were FACS (fluorescence-activated cell sorting) sorted from the spleens of 6- to 8-week-old C57BL/6 mice. FACS-sorted cells were activated with plate-coated anti-CD3 antibody (2 μg ml −1 ) and soluble anti-CD28 antibody (2 μg ml −1 ), and then induced to differentiate into T H 1 cells by supplementation with IL-12 (10 ng ml −1 ; Peprotech) plus anti-IL-4 antibody (11B11; BD Pharmingen), T H 2 cells with IL-4 (40 ng ml −1 ; Peprotech) plus anti-IFN-γ antibody (XMG1.2; BD Pharmingen), T H 17 differentiation, cells usually received anti-IL-4 and anti-IFN-γ plus a T H 17 ‘cocktail’, containing TGF-β1 (2 ng ml −1 ; R&D), IL-6 (30 ng ml −1 ; Peprotech), tumour necrosis factor (10 ng ml −1 ; Peprotech), IL-1β (10 ng ml −1 ; Peprotech) and IL-23 (20 ng ml −1 ; Peprotech), inducible Treg cells with TGF-β1 (5 ng ml −1 ; R&D) and recombinant mouse IL-2 (50 U ml −1 ; Peprotech). Neutralizing anti-IFN-γ and anti-IL-4 were both used at a concentration of 10 μg ml −1 . Cells stimulated under ‘neutral’ conditions (anti-IL-4 plus anti- IFN-γ, but no additional cytokines) were considered ‘T H 0’ cells. Intracellular staining and flow cytometry For intracellular cytokine staining, cells obtained from in vitro culture or from spleens or CNS infiltrates of mice with EAE were incubated in a tissue culture incubator for 5 h at 37 °C with phorbol 12-myristate 13-acetate (50 ng ml −1 ; Sigma), ionomycin (750 ng ml −1 ; Sigma) and brefeldin A (10 μg /ml −1 ; Sigma). Surface staining was performed as described above with the corresponding fluorescence-labelled surface antibodies. After surface staining, the cells were resuspended in fixation/permeabilization solution (Cytofix/Cytoperm Kit; BD Pharmingen), and intracellular cytokine staining was performed according to the manufacturer’s protocol. For Foxp3 staining, the cells were not stimulated with phorbol 12-myristate 13-acetate and ionomycin, instead the cells were stained according to the manufacturer’s protocol (Foxp3 Staining Buffer Set, eBioscience). FACS Calibur (BD Biosciences) and FlowJo software were used for analysis. Sample data were acquired by FACS Calibur cytometer (BD Biosciences) and analysed using FlowJo software. Transfer model of colitis Naive T cells (CD4 + CD25 − CD44 lo CD62L hi ) from C57BL/6 mice were sorted by FACS and then transferred into Rag1 –/– mice alone or in combination with CD4 + CD25 hi Treg cells. After T-cell reconstitution, the mice were weighed weekly and monitored for signs of disease. Mice were killed at 6 weeks after T-cell transfer and their colons were subjected to histopathological analysis. Epithelial cell hyperplasia and leukocyte infiltration were mainly evaluated. EAE The induction of EAE was described previously [49] , [50] . Briefly, C57BL/6 mice at 6–8 weeks of age were induced by a subcutaneous immunization in the back region with 300 μg of the MOG peptide (35–55) in Complete Freund’s Adjuvant (CFA; Difco). Pertussis toxin (List Biological Laboratories, Inc.) at a dose of 200 μg per mouse in PBS was administered intraveously on the day of immunization and once more 48 h later. The disease score was evaluated as previously described (ref. 49 ): 0, no clinical signs; 1, limp tail; 2, paraparesis (weakness, incomplete paralysis of one or two hind limbs); 3, paraplegia (complete paralysis of two hind limbs); 4, paraplegia with fore limb weakness or paralysis and 5, moribund state or death. For histology, spinal cords were removed from MOG-immunized mice and were immediately fixed in 4% paraformaldehyde. Paraffin-embedded 5-μm sections of spinal cord were stained with haematoxylin–eosin or Luxol Fast Blue and then examined by light microscopy. Quantitative PCR Total RNA was extracted from the cells and mouse tissues with TRIzol reagent (Invitrogen) according to the manufacturer’s instructions. cDNA was synthesized with PrimeScript RT reagent kit (Takara). The expression of the genes encoding mouse Foxp3, Tgfb1, Stat3, Rorc, Il17a, Il17f, Gata3, Il4, Il5, Il13, Ifng, Il21, Il22, Il23r and so on were quantified by real-time PCR using the SYBR Premix ExTaq kit (Takara) (sequence data are available upon request). All gene expression results were normalized to the expression of the housekeeping gene Rpl13a . Amplification of cDNA was performed on an AbiPrism 7900 HT cycler (Applied Biosystems). Mature miR-125a and other miRNAs were assayed with a specific TaqMan kit from Applied Biosystems, and their expression was normalized to the expression of snoRNA202 or RNU48. MiRNA agomir and antagomir MiR-125a agomir and antagomir were purchased from Ruibo Biotech. MiRNA agomirs are chemically synthesized dsRNA oligonucleotides used to mimic miRNA. The terminal nucleotides at both ends of the dsRNAs are modified by an O-methyl moiety at the 2′-ribose position. Another modification is cholesteryl functionality at the 5′ end of the RNA at sense strand. MiRNA antagomirs are single-stranded oligonucleotides used to silence endogenous miRNAs. Similarly, different chemical modifications are used to enhance the stability and cellular uptake, including partial phosphorothioate backbone modifications, fully 2′-OMe sugar modifications and 3′-cholesterol conjugation. Universal negative controls for both agomirs and antagomirs are based on the sequences of cel-miR-67 in Caenorhabditis elegans , which has been confirmed to have minimal sequence identity with miRNAs in human, mouse or rat. Luciferase assays For the 3′UTR reporter assay, psiCHECK-2 vector (Promega) was used to clone the 3′UTRs of all the predicted targets of miR-125a. Site-specific mutants were generated by PCR in psiCHECK-2 vector. HEK293T cells were seeded in the wells of a 96-well plate 1 day before transfection, and then each well was transfected with a mixture of 10 ng 3′UTR luciferase reporter vector and 0.5 μl of 20 μM miRNA agomirs. Twenty-four hours after transfection, the cells were lysed and the luciferase activity was measured. The ratio of renilla luciferase to firefly luciferase was calculated for each well. Immunoblots Lysates were resolved by electrophoresis, transferred to polyvinylidene fluoride (PVDF) membrane and probed with antibodies directed against Stat3 or Actin. Images have been cropped for presentation in Fig.6d . Full-size images are presented in Supplementary Fig.14 Statistics The nonparametric Mann–Whitney U -test was applied for the statistical comparison of health and patient samples. A two-tailed Student’s t -test was applied for statistical comparison of two groups or where appropriate. The one-way analysis of variance and least significant difference t -test was used for comparison of multiple groups. P values <0.05 were considered statistically significant. Accession codes : Array data are available in GEO under accession code GSE66608 . How to cite this article : Pan, W. et al. MiR-125a targets effector programs to stabilize Treg-mediated immune homeostasis. Nat. Commun. 6:7096 doi: 10.1038/ncomms8096 (2015).